Quantifying interface and bulk contributions to spin–orbit torque in magnetic bilayers Spin–orbit interaction-driven phenomena such as the spin Hall and Rashba effect in ferromagnetic/heavy metal bilayers enables efficient manipulation of the magnetization via electric current. However, the underlying mechanism for the spin–orbit interaction-driven phenomena remains unsettled. Here we develop a sensitive spin–orbit torque magnetometer based on the magneto-optic Kerr effect that measures the spin–orbit torque vectors for cobalt iron boron/platinum bilayers over a wide thickness range. We observe that the Slonczewski-like torque inversely scales with the ferromagnet thickness, and the field-like torque has a threshold effect that appears only when the ferromagnetic layer is thinner than 1 nm. Through a thickness-dependence study with an additional copper insertion layer at the interface, we conclude that the dominant mechanism for the spin–orbit interaction-driven phenomena in this system is the spin Hall effect. However, there is also a distinct interface contribution, which may be because of the Rashba effect. Local electrical manipulation of magnetization is a promising candidate for information storage and processing owing to the switching reliability and its easy large-scale integration [1] , [2] , [3] , [4] . One way to realize electrical control of magnetization is to leverage the spin–orbit interaction (SOI), through which an electric current exerts an effective field and torque on the magnetization [5] , [6] . In recent years, electric-current-induced magnetization switching in heavy metal (HM)/ferromagnetic metal (FM) bilayers has attracted great attention because of its high efficiency in magnetization switching, architectural simplicity and potential to couple with voltage-controlled magnetic anisotropy [7] , [8] . Besides magnetization switching, the SOI effect also provides a convenient tool to manipulate magnetic domains [9] , [10] , [11] , [12] , [13] . Although these beneficial effects have been successfully demonstrated, researchers are still debating the underlying principle, as to whether the dominating SOI arises from the HM/FM interface due to the Rashba effect or from the bulk of the HM due to the spin Hall effect. It has been theoretically predicted that both the Rashba effect and the spin Hall effect generate, with only quantitative differences [14] , a spin–orbit effective field (SOF) and spin–orbit-effective Slonczewski-like torque (SOT) on the magnetization. Several experimental techniques have been developed to quantify the SOF and SOT under a small electric current bias [15] , [16] . However, these techniques are limited to thin films with perpendicular anisotropy. Here, we develop a magneto-optic Kerr effect (MOKE)-based spin–orbit torque magnetometer that sensitively detects the SOT and SOF. Combined with more sensitive SOF detection via the planar Hall effect (PHE) [17] , we obtain the thickness dependence of SOT and SOF over a wide range of FM thicknesses. On the basis of this technique, we are also able to quantitatively determine the bulk and interface contributions to the overall SOI effect. Current-induced magnetization reorientation Despite the different SOI origins of the interface Rashba effect and the spin Hall effect, the SOF and SOT generated from a current through the HM/FM bilayer can be described by the Landau–Lifshitz–Gilbert–Slonczewski equation, where is the normalized magnetization vector, γ is the gyromagnetic ratio, μ 0 is the permeability of vacuum, is the total effective field including the external field , anisotropy field and Oersted field generated from the current, α is the damping coefficient, is the unit vector that is in-plane and orthogonal to the electric current, and and describe the SOF and SOT, respectively. In order to determine the magnitude of and , it is desirable to analyse the linear response of the magnetization vector in a saturated magnetization state to a small electric current. In this case, the magnetization is uniform and the Dzyaloshinskii–Moriya interaction can be neglected [18] . In a simplified scenario shown in Fig. 1a , where the magnetization of the FM layer is uniformly saturated in the film plane by an external field and an electric current is applied in the same direction, the effect from the SOI can be viewed as an in-plane effective field and an out-of-plane effective field (ref. 17 ). 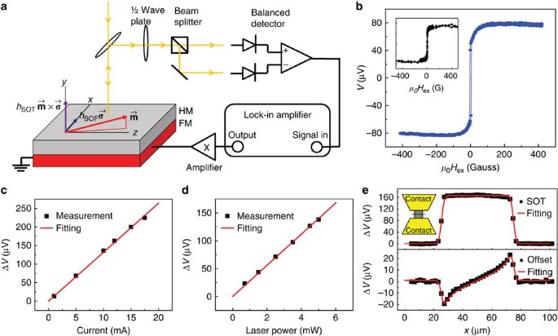Figure 1: SOT detected with the polar MOKE. (a) Experimental setup for using polar MOKE to detect the SOT. A lock-in amplifier supplies an ac current through the sample along thezdirection, which generates SOF and SOT that rotate the magnetization in-plane and out-of-plane from thexzplane, respectively. The reflected laser polarization changes with the magnetization of the sample because of the MOKE. The change in the polarization is converted to a voltage signal through a series of optical components and a balanced detector. The voltage signal is detected by the same lock-in amplifier. (b) An example experimental result from CoFeB/Pt with a 12 mA bias current and 5 mW laser power. The inset is the magnetization hysteresis of the same sample. (c) The linear bias current dependence of the MOKE response. The laser power is kept at 5 mW with a beam radius of 2 μm, which corresponds to a power density of 4 × 108W m−2. (d) The linear laser power dependence of the MOKE response. The bias current is kept at 10 mA, which corresponds to a current density of 4 × 1010A m−2. (e) Determination of the magnitude of the SOT using self-calibration. MOKE voltages are measured as the laser position is held fixed and the sample is moved along thexdirection. The bias current is 12 mA. The magnitude of the SOT is determined to beβ=1.83±0.7 nm by fitting both MOKE voltage curves because of the SOT and out-of-plane Oersted field. This results in a current-induced magnetization reorientation Figure 1: SOT detected with the polar MOKE. ( a ) Experimental setup for using polar MOKE to detect the SOT. A lock-in amplifier supplies an ac current through the sample along the z direction, which generates SOF and SOT that rotate the magnetization in-plane and out-of-plane from the xz plane, respectively. The reflected laser polarization changes with the magnetization of the sample because of the MOKE. The change in the polarization is converted to a voltage signal through a series of optical components and a balanced detector. The voltage signal is detected by the same lock-in amplifier. ( b ) An example experimental result from CoFeB/Pt with a 12 mA bias current and 5 mW laser power. The inset is the magnetization hysteresis of the same sample. ( c ) The linear bias current dependence of the MOKE response. The laser power is kept at 5 mW with a beam radius of 2 μm, which corresponds to a power density of 4 × 10 8 W m −2 . ( d ) The linear laser power dependence of the MOKE response. The bias current is kept at 10 mA, which corresponds to a current density of 4 × 10 10 A m −2 . ( e ) Determination of the magnitude of the SOT using self-calibration. MOKE voltages are measured as the laser position is held fixed and the sample is moved along the x direction. The bias current is 12 mA. The magnitude of the SOT is determined to be β =1.83±0.7 nm by fitting both MOKE voltage curves because of the SOT and out-of-plane Oersted field. Full size image where arises from the demagnetizing effect, where M s is the saturation magnetization and K ⊥ is the surface anisotropy energy density, and and are the in-plane and out-of-plane current-induced fields due to Ampere’s law, respectively. By detecting the amount of current-driven magnetization reorientation, the SOF and SOT can be determined. Detection of SOT and SOF It is well known that MOKE microscopy can selectively detect each component of the magnetization by varying the incidence angle of the laser [19] . In particular, when the laser is incident normal to the surface, the laser polarization is only sensitive to the perpendicular magnetization (polar MOKE), making it an ideal technique to detect the out-of-plane magnetization reorientation and hence the effect of the SOT. The experiment setup is shown in Fig. 1a . The HM/FM bilayer is patterned into a 50 μm × 50 μm strip. When an alternating current I ac is applied to the strip, the out-of-plane magnetization Δ m y of the FM changes based on equation (2), causing the polarization of the reflected laser to rotate because of the MOKE. The reflected laser is sent through polarization optics to a balanced detector, which outputs a voltage V that is proportional to the polarization rotation of the laser. Since the SOT and SOF are both proportional to the current, V is proportional to the applied current I ac and can be measured by a lock-in amplifier. Figure 1b shows an example result using Ti(1)/Co 40 Fe 40 B 20 (0.85)/Pt(5), where the numbers in parentheses are thicknesses in nanometres. The curve resembles the magnetization hysteresis of the sample shown in the inset, consistent with equation (2), since switches sign as the magnetization switches and M eff is much greater than the external field applied. On the other hand, remains a constant, which raises the entire curve vertically. Figure 1c,d shows the linear responses to the bias current and laser power, which rules out contributions from thermal effects. The magnitude of the SOT is determined through a self-calibration method. We perform a line scan by keeping the laser position fixed and translating the sample along the x direction. The MOKE voltages at the positive saturation field V [+ H ex ] and negative saturation field V [− H ex ] are taken. The voltage signal corresponding to the SOT and the out-of-plane Oersted field can be extracted, respectively. Therefore, the magnitude of the SOT can be correlated with the out-of-plane Oersted field, and the latter is readily solvable using Ampere’s law: The SOT is determined by fitting the line scan, which is discussed in detail in the Methods section. In this sample the applied current is 12 mA. Since the resistivities of Ti and Co 40 Fe 40 B 20 (hereafter CoFeB) are much greater than that of Pt, as shown in the Methods section, we estimate that all of the current flows through the Pt layer, giving rise to a current density of j Pt =4.8 × 10 10 A m −2 . We then determine the material-related SOT coefficient β T = h SOT / j Pt =1.83±0.7 nm. By assuming that the SOT is contributed by the spin Hall effect and using the equation proposed by Ando et al . [20] and Liu et al . [21] , , we determine a spin Hall angle of 0.076±0.007 for Pt, which is similar to reported results [20] , [21] . Here the parameters used are μ 0 M s =1.6 T and d CoFeB =0.85±0.05 nm. MOKE can also detect the in-plane magnetization with oblique angle incidence and therefore determine the SOF as described in the Methods section. However, in this manuscript, we choose to use the second-order PHE method to measure the SOF because of its better sensitivity [17] . As shown in Fig. 2a , the sample is electrically detected in a Hall bar structure with in-plane magnetization orientation. The second-order planar Hall voltage is taken at various small transverse magnetic fields for the purpose of calibration, Δ V ( h cal )= V (+ I, + h cal , H ex )+ V (− I ,− h cal , H ex ), where I is the applied current and h cal is the applied calibration field. 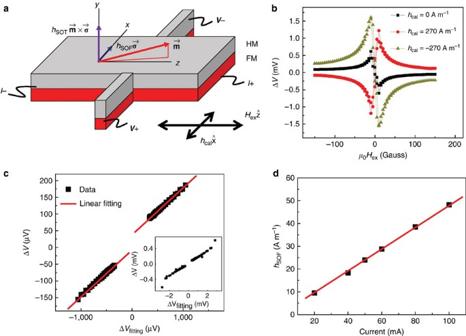Figure 2: SOF detected with the second-order PHE method. (a) Experimental setup for using the second-order PHE to detect the in-plane magnetization reorientation and the SOF. A transverse fieldhcalis applied to calibrate the response of the second-order PHE voltage in order to quantify the SOF. (b) Example measured second-order PHE curve of the Ti(1)/CoFeB(0.75)/Pt(5) under several calibration field strengths. The applied dc current is 50 mA. (c) Linear regression algorithm to extract the SOF. Thexaxis is obtained by ΔVFitting=ΔV(hcal=−270 A m−1)−ΔV(hcal=270 A m−1), and theyaxis is ΔV(hcal=0 A m−1) at the corresponding magnetic field. The positively saturated data and negatively saturated data are fitted separately with the average slope taken as the ratio between the total current-induced field and the calibration field. The inset shows the overall curve at both saturated and unsaturated fields. (d) The linear bias current dependence of the SOF indicates that the measurement is still in the linear regime. Under the small perturbation limit, the second-order PHE voltage Δ V is linearly proportional to the current-induced magnetization reorientation Δ m x as calculated in equation (2) and is therefore proportional to the transverse field including the SOF, in-plane Oersted field and calibration field h cal , Figure 2: SOF detected with the second-order PHE method. ( a ) Experimental setup for using the second-order PHE to detect the in-plane magnetization reorientation and the SOF. A transverse field h cal is applied to calibrate the response of the second-order PHE voltage in order to quantify the SOF. ( b ) Example measured second-order PHE curve of the Ti(1)/CoFeB(0.75)/Pt(5) under several calibration field strengths. The applied dc current is 50 mA. ( c ) Linear regression algorithm to extract the SOF. The x axis is obtained by Δ V Fitting =Δ V ( h cal =−270 A m −1 )−Δ V ( h cal =270 A m −1 ), and the y axis is Δ V ( h cal =0 A m −1 ) at the corresponding magnetic field. The positively saturated data and negatively saturated data are fitted separately with the average slope taken as the ratio between the total current-induced field and the calibration field. The inset shows the overall curve at both saturated and unsaturated fields. ( d ) The linear bias current dependence of the SOF indicates that the measurement is still in the linear regime. Full size image The second-order PHE voltage curves with different calibration fields are shown in Fig. 2b . The curves have a similar profile with different magnitudes. The SOF can be extracted by comparing Δ V ( h cal =0 A m −1 ) and Δ V ( h cal =−270 A m −1 )−Δ V ( h cal =270 A m −1 ) using a linear regression algorithm, as shown in Fig. 2c . Here the data at magnetic fields <30 Gauss are not included in the fitting to satisfy the requirement of small angle perturbation. The data at positively saturated state and negatively saturated state are fitted separately with the slope being =0.137±0.002. An offset between the two linear fittings can be observed, which corresponds to the thermal effect and anomalous Hall effect because of out-of-plane magnetization reorientation [17] . By assuming most of the current flows through the Pt layer, we can calculate the SOF by subtracting the in-plane Oersted field =50 A m −1 , where w =500 μm is the width of the Hall bar and I =50 mA. The SOF of Ti(1)/CoFeB(0.75)/Pt(5) is extracted to be 24.0±1.1 A m −1 at a current density of 2 × 10 10 A m −2 through the Pt. We similarly determine the SOF coefficient =1.20±0.05 nm. A consistent result is obtained using longitudinal MOKE as shown in the Methods section. Figure 2d shows the linear dependence of the SOF on the bias current applied, suggesting that the measurement is in the linear response regime. FM thickness-dependence study We measure the magnitude of the SOT and SOF for a series of samples Ti(1)/CoFeB( x )/Pt(5), where x spans from nominal 0.65 to 5.75 nm. The addition of Ti is for better adhesion and continuity of the ultrathin CoFeB layer. Adding the Ti layer does not introduce significant SOI because of its high resistivity and low atomic number. This is confirmed by a control sample of Ti(1)/CoFeB(0.95)/Cu(5) as shown in Supplementary Fig. 1 . As shown in Fig. 3a and its inset, the SOT coefficient follows the 1/ d CoFeB dependence and monotonically increases when the CoFeB gets thinner. On the other hand, the thickness dependence of the SOF coefficient shows a threshold effect that remains near zero for thick CoFeB but increases rapidly when the CoFeB is thinner than 1 nm. Haney et al . [14] computed the dependence of SOF and SOT on the thickness of the FM based on the Boltzmann equation considering both the bulk spin Hall effect in the HM and the Rashba effect at the FM/HM interface. The Boltzmann model calculations showed that the bulk spin Hall effect results in a constant scaled SOT ( Fig. 6a of Haney et al . [14] ), which corresponds to a 1/ d CoFeB dependence. The calculated Rashba effect results in a decreasing scaled SOT with decreasing FM thickness, corresponding to a much faster decay than the 1/ d CoFeB dependence in the absolute SOT. This suggests that our results are consistent with the spin Hall effect mechanism rather than the Rashba effect mechanism. In the context of the spin Hall effect, the sharp increase in the SOF for very thin FMs may be understood by the finite spin-dephasing length of the FM. In other words, this result is in accordance with the spin-dephasing effect in the spin torque transfer process [22] , [23] , where the spin Hall-induced spin current undergoes a Larmor precession because of the exchange interaction with the local magnetization. When the CoFeB is thinner than a characteristic spin-dephasing length, an effective magnetic field can be generated on the magnetization from the spin torque transfer process. Kim et al . [15] have recently performed a study of the SOT and SOF in a Ta/CoFeB/MgO system with perpendicular geometry [15] . Their result on the SOF also shows a monotonic increase with the reduction of CoFeB thickness. However, the sign of the SOF is opposite to what one would expect from the spin Hall effect. Their result of the SOT dependence on the CoFeB thickness is also different from what we measured. This may indicate that the dominant mechanism determining spin–orbit torques is different for different structures. 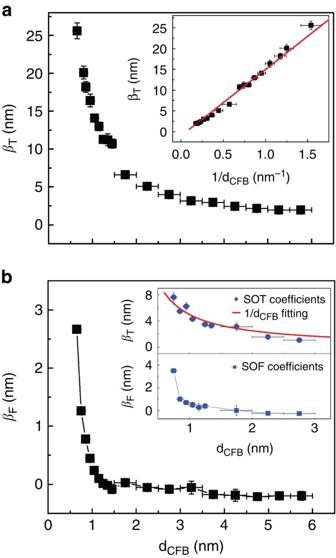Figure 3: Quantification of the SOT and SOF coefficients. (a). Measured SOT coefficient of Ti(1)/CoFeB(x)/Pt(5), wherexspans from nominal 0.65 to 5.75 nm. The inset shows the 1/dCoFeBdependence of the SOT coefficients. Here the error bar of theyaxis is obtained from the linear regression, as discussed in the Methods section. The error bar of thexaxis is because of possible misalignment in fabricating the wedge-shaped sample, as described in the Methods section. (b) Measured SOF coefficient of the same series of samples as ina. The SOF remains nearly zero when the CoFeB is thick and increases rapidly as the CoFeB becomes thinner than 1 nm. The inset shows the SOT and SOF of Ti(1)/CoFeB(x)/Cu(2)/Pt(5), where the direct interface between CoFeB and Pt is removed. Figure 3: Quantification of the SOT and SOF coefficients. ( a ). Measured SOT coefficient of Ti(1)/CoFeB( x )/Pt(5), where x spans from nominal 0.65 to 5.75 nm. The inset shows the 1/ d CoFeB dependence of the SOT coefficients. Here the error bar of the y axis is obtained from the linear regression, as discussed in the Methods section. The error bar of the x axis is because of possible misalignment in fabricating the wedge-shaped sample, as described in the Methods section. ( b ) Measured SOF coefficient of the same series of samples as in a . The SOF remains nearly zero when the CoFeB is thick and increases rapidly as the CoFeB becomes thinner than 1 nm. The inset shows the SOT and SOF of Ti(1)/CoFeB(x)/Cu(2)/Pt(5), where the direct interface between CoFeB and Pt is removed. Full size image Figure 6: Extraction of the SOF coefficient from longitudinal MOKE. ( a ) Experimental setup for using longitudinal MOKE to detect the SOF. 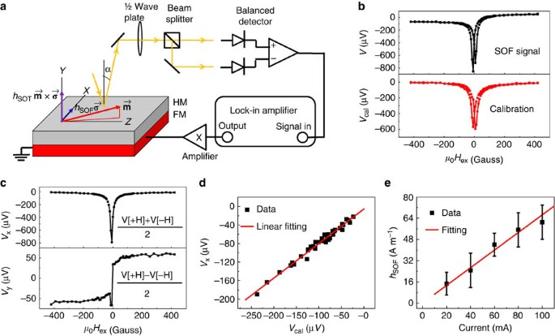Figure 6: Extraction of the SOF coefficient from longitudinal MOKE. (a) Experimental setup for using longitudinal MOKE to detect the SOF. The setup is identical with the polar MOKE shown inFig. 1a, except that the laser is obliquely incident on the sample in thexyplane. The incident angle is set to be about 20°. (b) Measured voltage from the lock-in amplifier when passing an ac current 100 mA through the sample (500 μm in width) is shown in the top curve. The curve is asymmetric owing to the out-of-plane magnetization reorientation because of the SOT. The calibration is performed by applying an ac current through a metallic wire behind the sample, which generates an Oersted field (216±8 A m−1) that drives the in-plane magnetization reorientation. As shown in the lower graph, the curve is symmetric since the calibration field has no torque-like term. (c) The magnetization reorientation because of the SOF (top curve) and SOT (bottom curve) can be separated by their different symmetries. (d) The magnitude of the SOF is extracted using a linear regression algorithm by comparing the top curve inFig. 2cand the calibration curve inFig. 2b. Only data between 50 and 300 Gauss are used in the fitting, where the magnetization is well saturated. In this example fitting, the ratio between the current-induced effective field and the calibration field is 0.74±0.03, which gives rise to a current-induced field of 160±16 A m−1. After removing the 104 A m−1Oersted field generated by the current, we obtain ahSOF=56±16 A m−1. (e) The extracted SOF is linearly proportional to the bias current, suggesting that the measurement is still in the linear regime. The setup is identical with the polar MOKE shown in Fig. 1a , except that the laser is obliquely incident on the sample in the xy plane. The incident angle is set to be about 20°. ( b ) Measured voltage from the lock-in amplifier when passing an ac current 100 mA through the sample (500 μm in width) is shown in the top curve. The curve is asymmetric owing to the out-of-plane magnetization reorientation because of the SOT. The calibration is performed by applying an ac current through a metallic wire behind the sample, which generates an Oersted field (216±8 A m −1 ) that drives the in-plane magnetization reorientation. As shown in the lower graph, the curve is symmetric since the calibration field has no torque-like term. ( c ) The magnetization reorientation because of the SOF (top curve) and SOT (bottom curve) can be separated by their different symmetries. ( d ) The magnitude of the SOF is extracted using a linear regression algorithm by comparing the top curve in Fig. 2c and the calibration curve in Fig. 2b . Only data between 50 and 300 Gauss are used in the fitting, where the magnetization is well saturated. In this example fitting, the ratio between the current-induced effective field and the calibration field is 0.74±0.03, which gives rise to a current-induced field of 160±16 A m −1 . After removing the 104 A m −1 Oersted field generated by the current, we obtain a h SOF =56±16 A m −1 . ( e ) The extracted SOF is linearly proportional to the bias current, suggesting that the measurement is still in the linear regime. Full size image Although the results shown in Fig. 3 imply that the dominant mechanism of spin–orbit torque in this bilayer is the bulk spin Hall effect, one has to quantify the interface effect separately from the bulk effect in order to be conclusive. To this purpose, we further perform the same study on a series of samples of Ti(1)/CoFeB( x )/Cu(2)/Pt(5), where the 2-nm Cu removes the possible CoFeB/Pt interface effect without significantly reducing the spin current because of its weak spin–orbit coupling. We estimate the effective SOT and SOF coefficients in Ti(1)/CoFeB( x )/Cu(2)/Pt(5) by assuming that all currents flow through the Pt, which overestimates the current density and therefore would result in reduced values compared with those of the Ti(1)/CoFeB( x )/Pt(5) sample. As shown in the inset of Fig. 2b , similar trends of the SOT and SOF are observed, which asserts the primary contribution of the spin Hall effect to the SOT and SOF. However, the ratio of the magnitude in the SOT and SOF coefficients is different between the samples with and without Cu, implying that there may be subtleties at the CoFeB/Pt interface. Therefore, we performed more systematic study by varying the Cu layer thickness as shown below. Determination of interface contribution Both the Rashba effect and the spin Hall effect can produce the SOF and SOT [14] , [24] , [25] , [26] . The difference between the two effects depends quantitatively on the Rashba coefficient, spin Hall angle, spin-dephasing length and even the current distribution between the layers [14] . However, the determination of these parameters has not been well-established and variations in these parameters may lead to different conclusions. Here we treat the controversy in a different way by separating the contribution due to the interface from that due to nonlocal effects mediated by spin current. By inserting a thin Cu layer in between CoFeB and Pt, the direct interface effect is removed. Therefore, the SOT and SOF detected in the Ti(1)/CoFeB(0.7)/Cu(x)/Pt(5) samples are only because of nonlocal effects, where the SOI occurs in either the bulk of the Pt because of the spin Hall effect or the Cu/Pt interface, and the spin current diffuses into the CoFeB through the almost dissipationless Cu layer. In this case, despite the different current distributions because of the varying thicknesses of Cu, the ratio between the SOT and SOF h SOT / h SOF should remain the same as long as the Cu layer is thick enough to isolate the direct interface effect between the CoFeB and Pt. If the CoFeB/Pt interface makes a significant contribution to the SOF and SOT, one should observe a deviation of h SOT / h SOF when the Cu layer is removed. The experimental data are shown in Fig. 4a . The SOF increases slightly with the insertion of a very thin Cu layer and reduces with increasing Cu thickness, while the SOT exhibits a monotonic decay with Cu thickness. The overall reduction in the SOF and SOT is mainly because the Cu partially shorts the current through the Pt. Another possible effect is that the Cu/CoFeB interface may have a different spin-mixing conductance than the Pt/CoFeB interface, resulting in a different spin transfer torque efficiency [27] , [28] . Despite the significant reduction in both SOF and SOT, the ratio between the two remains near 0.2 when the Cu is thicker than 0.75 nm, as shown in Fig. 4b . This suggests that both the SOF and SOT have the same origin of nonlocal spin current. However, when the Cu is thinner than 0.75 nm, this ratio is lower than 0.2, indicating the existence of an interface effect. This interface effect may arise from the Rashba effect. Since the Rashba effect tends to produce a much larger effective field than torque, it is reasonable to estimate that the SOT arises mostly from the spin Hall effect. Therefore, the pure spin Hall-induced effective field is estimated from the SOT to be β F_spin Hall = β T_spin Hall × 0.2=4.4 nm assuming the same SOF/SOT ratio as samples with Cu inserted. The Rashba field contribution with no Cu insertion is then estimated to be β F_Rashba = β F − β F_spin Hall =−2.4 nm. We similarly perform a SOF measurement study on the Ti(1)/Ni 80 Fe 20 (1.5)/Cu(0-5)/Pt(5) system. Although the magnitude of the SOF is comparable to that of the Ti(1)/ CoFeB(0.7)/Cu(0–5)//Pt(5), we observe monotonic decay of the SOF with Cu insertion that differs from the samples using CoFeB. We speculate a correlation between the interface SOI and possible hybridization between Co and Pt [29] . In other words, the hybridization between Ni (or Fe) and Pt might be much weaker than that between Co and Pt so that no distinct interface effect is observed in Ni 80 Fe 20 /Pt samples. It should be pointed out that the Rashba effect is not the only explanation for the reduction in the SOF with direct contact of CoFeB and Pt. Another possible reason is the proximity effect [30] , in which the interface of the Pt may become magnetic and effectively increase the thickness of the FM layer. Consequently, both the SOF and SOT decrease. 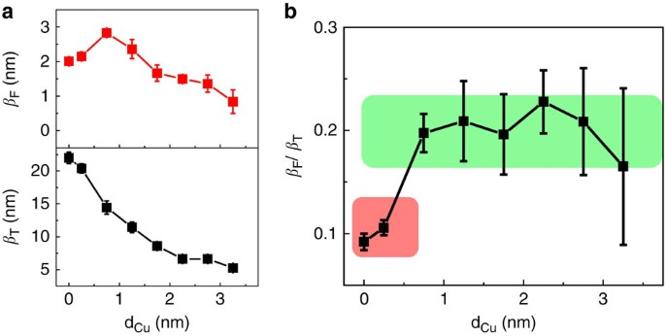Since the SOF decreases more rapidly than the SOT as the FM thickness increases, the ratio between the two decreases when the proximity effect effectively increases the thickness of the FM layer. Figure 4: Observation of the interface contribution. (a) Measured SOF and SOT coefficients in Ti(1)/CoFeB(0.7)/Cu(x)/Pt(5). The SOF coefficient shows an increase with very thin copper insertion and then decrease as the copper layer gets thicker, while the SOT coefficient shows a monotonic decay with increasing copper layer thickness. (b) The ratio between the SOF and SOT coefficients manifests two regimes as highlighted in the graph. In the green regime, where copper is thick enough to remove the interface effect between CoFeB and Pt, the βF/βTvalues are near 0.2. In the red regime, where the copper is too thin to form a continuous film, theβF/βTis lower, suggesting that there exists an interface effect that produces a SOF and SOT based on a different mechanism from the effect of the nonlocal spin current. Figure 4: Observation of the interface contribution. ( a ) Measured SOF and SOT coefficients in Ti(1)/CoFeB(0.7)/Cu( x )/Pt(5). The SOF coefficient shows an increase with very thin copper insertion and then decrease as the copper layer gets thicker, while the SOT coefficient shows a monotonic decay with increasing copper layer thickness. ( b ) The ratio between the SOF and SOT coefficients manifests two regimes as highlighted in the graph. In the green regime, where copper is thick enough to remove the interface effect between CoFeB and Pt, the β F /β T values are near 0.2. In the red regime, where the copper is too thin to form a continuous film, the β F / β T is lower, suggesting that there exists an interface effect that produces a SOF and SOT based on a different mechanism from the effect of the nonlocal spin current. Full size image Our experiment has several important implications. The fact that both SOT and SOF persist even with the insertion of a copper layer indicates that the spin Hall effect contributes to both the SOT and SOF. However, there is an important interface effect at the Pt/CoFeB interface that contributes additional SOT and SOF. This implies that another way to harness the spin–orbit-interaction-induced magnetization switching is by engineering the interface. It should be emphasized that, although the spin Hall effect dominates the CoFeB/Pt system under this study, other systems with stronger interface SOI may be more influenced by the Rashba effect. The development of the spin–orbit torque magnetometer together with the Cu insertion method to isolate the interface allows quantitative determination of bulk and interface contributions in various systems. Sample fabrication The samples were deposited via magnetron sputtering. The deposition rates were 0.13 nm s −1 (Cu) and 0.07 nm s −1 (Ti, Pt and Co 40 Fe 40 B 20 ) in an argon pressure of 4.5 × 10 −3 Torr. The resistivities of these films measured at 10 nm are, respectively, ρ Cu (71.2 nΩm)< ρ Pt (211.8 nΩm)<< ρ CoFeB (2,249.6 nΩm)<< ρ Ti (19,632 nΩm). The samples for thickness-dependence studies are fabricated by offsetting the sample (4 cm long) during sputtering. The thickness is extracted based on the position of the sample. Since the offset has a 2-mm error, the determination of the thickness has an error of 5% of the entire wedge thickness. The relative thickness among the wedges should be accurate. Therefore, no thickness error is added in Fig. 4 for clarity of the graph. The samples used for the SOT measurements were lithographically patterned into 50 μm × 50 μm squares connected by two contact pads consisting of Ti(5)/Cu(200)/Au(50). The samples used for the SOF measurements were patterned into Hall bar structures 500 μm wide and 3 mm long. The contact pads of the Hall bars are capped with Ti(5)/Cu(200)/Au(50). Setup of MOKE measurement The laser source used for the MOKE measurement is a mode-locked Ti:Sapphire laser working at 725 nm centre wavelength. For the SOT measurement with normal incidence, a × 20 objective is used to focus the laser on the sample and collimate the reflected beam. The error of the incidence angle is better than 0.1°. For the SOF measurement with oblique incidence, the same sample with the Hall bar structure used for the second PHE measurement is used. In this case, two lenses are used to focus and collimate the laser. The incidence angle is set to be about 20°. The calibration field is applied by applying an ac electric current (1 A) through a flat wire (1 mm wide and 1 cm long) underneath the sample. The distance from the sample to the wire is about 650±50 μm. The radiated field is calculated to be 216±8 A m −1 . Extraction of SOT from polar MOKE For a magnetic thin film with width w and thickness d , where d << w , the out-of-plane Oersted field distribution generated by an electric current flowing through the magnetic thin film is given by where I c is the total electric current flowing through the film and x ∈ [0, w ] is the position perpendicular to the current direction. For the small field limit, the magnetization reorientation because of the current-induced out-of-plane Oersted field is given as where H ex is the external field and M eff is the effective magnetization. It should be noted that in this derivation, we consider the magnetization reorientation only to be because of the local Oersted field by neglecting the exchange coupling between the nearest neighbours. This is a reasonable assumption, since both the magnitude and gradient of the magnetic field are weak and the exchange energy is estimated to be six orders smaller than the Zeeman energy. Owing to the finite size of the laser spot, the response of the Kerr rotation is calculated as the integration of the local magnetization reorientation weighted by the Gaussian function that describes the spatial distribution of the laser. where r is the radius of the laser spot and η describes the sensitivity of MOKE response: η= V MOKE /Δ m y . Similarly, the MOKE response because of the SOT-induced magnetization reorientation can be derived as where h SOT is uniform over the sample but switches sign when the magnetization switches. By moving the sample along the x direction with a motion stage, the laser beam scans through the sample along its middle section. An example curve is shown in Fig. 5a,c using Ti(1)/Co 40 Fe 40 B 20 (0.85)/Pt(5). We then numerically simulated the curves based on equation(8) and equation (9), also shown in Fig. 5a,c . Here the unknown parameter is the starting position of the line scan, which can be obtained by aligning the experimental result and the fitting data. We then perform a linear regression algorithm on the experimental data and the corresponding simulation data to obtain the ratio between the two as shown in Fig. 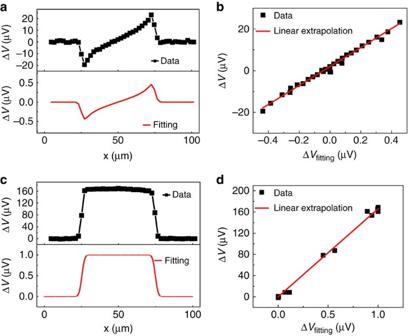5b,d . Figure 5: Extraction of the SOT coefficient from polar MOKE. The extraction is for the data shown inFig. 1e. (a) Measured offset of line scan ΔV=V[+H,x]+V[−H,x] and the corresponding fitting curve based on equation (8). (b) By plotting the fitting curve and the measured data together, the parameters in equation (8) can be calibrated from linear fitting. In this example curve, the parameter is given asηIc/w=45.5±1.2 μV. (c) Measured SOT signal of line scan ΔV=V[+H,x]−V[−H,x] and the corresponding fitting curve based on equation (9). (d) Linear extrapolation gives the parameter of SOT asηhSOT=166±3 μV. Therefore, the SOT coefficient is determined as=1.83±0.7 nm. The magnitude of the SOT is then calculated as Figure 5: Extraction of the SOT coefficient from polar MOKE. The extraction is for the data shown in Fig. 1e . ( a ) Measured offset of line scan Δ V = V [+ H , x ]+ V [− H , x ] and the corresponding fitting curve based on equation (8). ( b ) By plotting the fitting curve and the measured data together, the parameters in equation (8) can be calibrated from linear fitting. In this example curve, the parameter is given as ηI c / w =45.5±1.2 μ V . ( c ) Measured SOT signal of line scan Δ V = V [+ H , x ]− V [− H , x ] and the corresponding fitting curve based on equation (9). ( d ) Linear extrapolation gives the parameter of SOT as ηh SOT =166±3 μ V . Therefore, the SOT coefficient is determined as =1.83±0.7 nm. Full size image Supplementary Fig. 1 shows line scan curves for three samples: Ti(1)/CoFeB(0.75)/Pt(5), Ti(1)/CoFeB(0.95)/Cu(5) and Ti(1)/CoFeB(2)/Ta(5). The Pt(5) and Ta(5) samples have opposite spin Hall angle and hence opposite-sign SOT line scan curves but same out-of-plane Oersted field line scan curves. Cu(5) has a similar out-of-plane Oersted field line scan curve but a nearly 100 times weaker SOT line scan curve, which agrees with the weak SOI in Cu. These results show the high sensitivity and universality of the technique. Owing to the fine resolution of this optical method, it is also possible to obtain a spin–orbit torque landscape. As shown in Supplementary Fig. 2 , two-dimensional (2D) images of the out-of-plane magnetization reorientation because of the SOT and Oersted field can be obtained. Reasonable uniformity is observed near the centre of the sample. Extraction of SOF from longitudinal MOKE Similar to the polar MOKE with normal incidence, the longitudinal MOKE with oblique incidence is sensitive to the in-plane magnetization reorientation , as shown in Fig. 6a . Owing to the nature of the oblique incidence setup, it is inevitable that signals because of the out-of-plane reorientation also contribute: V = V x + V y , where V x Δ m x and V y Δ m y . However, we are able to separate V x from V y based on their different symmetries; that is, the component V x because of the SOF and in-plane Oersted field is symmetric at positive and negative external fields, while the component V y because of the SOT switches sign when the magnetization switches. Moreover, the V y because of the out-of-plane Oersted field can be viewed as constant background for thin magnetic films, as can be understood from equation (2). Therefore, we extract V x by . We also perform a calibration measurement by applying an ac magnetic field h cal in the x direction. In this case, the longitudinal MOKE signal V cal only corresponds to the in-plane magnetization rotation and is therefore symmetric, as shown in the inset of Fig. 6b . The SOF can be derived from using linear regression as shown in Fig. 6d . In the extrapolation, only data at saturated magnetization states are used. The extracted total current-induced field is 160±16 A m −1 at 100 mA bias, which is consistent with the 74.0±1.1 A m −1 at 50 mA bias extracted from the PHE method. However, the error of the oblique-incidence MOKE is typically higher than that extracted from the PHE method. It is speculated that the major source of error comes from the fact that the oblique-incidence MOKE has a less tight focus than the normal-incidence MOKE and is therefore more susceptible to environmental vibrations. Therefore, in this research we choose the more sensitive PHE method over the oblique-incidence MOKE method. In principle, both methods can be applied to measure the SOF. How to cite this article: Fan, X. et al . Quantifying interface and bulk contributions to spin–orbit torque in magnetic bilayers. Nat. Commun. 5:3042 doi: 10.1038/ncomms4042 (2014).